Evolution of the human-specific microRNA miR-941 MicroRNA-mediated gene regulation is important in many physiological processes. Here we explore the roles of a microRNA, miR-941, in human evolution. We find that miR-941 emerged de novo in the human lineage, between six and one million years ago, from an evolutionarily volatile tandem repeat sequence. Its copy-number remains polymorphic in humans and shows a trend for decreasing copy-number with migration out of Africa. Emergence of miR-941 was accompanied by accelerated loss of miR-941-binding sites, presumably to escape regulation. We further show that miR-941 is highly expressed in pluripotent cells, repressed upon differentiation and preferentially targets genes in hedgehog- and insulin-signalling pathways, thus suggesting roles in cellular differentiation. Human-specific effects of miR-941 regulation are detectable in the brain and affect genes involved in neurotransmitter signalling. Taken together, these results implicate miR-941 in human evolution, and provide an example of rapid regulatory evolution in the human linage. Gene expression changes are thought to be one of the main underlying causes of phenotypic differences between species, including human-specific features such as language, tool-making and much extended lifespan [1] . Mutations affecting the expression or structure of regulatory factors, such as transcription factors (TFs) and microRNAs (miRNAs), could result in misregulation of hundreds of genes and thus represent one of the powerful potential mechanisms of human expression evolution [2] . Previous studies focusing on TFs have indicated an excess of human-specific expression divergence for TFs in the liver [3] and the brain [4] . These findings suggest that changes in TF expression might explain some of the human-specific gene expression divergence. More recently, human-specific changes in transcript abundance during postnatal brain development were correlated with changes in miRNA expression [5] . This study further demonstrated that changes in the expression of transcriptional regulators influencing developmental trajectories of many genes in a synergistic fashion might have had a more pronounced effect on human brain development than changes affecting expression of single genes. Although the relevance of such regulatory changes to the evolution of human phenotypes remains to be determined, changes in miRNA expression might have had a notable role in driving gene expression divergence between human and chimpanzee brains [6] . In this study, we investigated the birth of novel miRNAs in the human lineage and their potential contribution to human-specific gene expression divergence. miRNAs are short (20–24 nucleotide) endogenous single-stranded RNAs involved in post-transcriptional gene silencing [7] . In mammals, mature miRNAs are processed from stable hairpin structures by Drosha and Dicer endonucleases. Mature miRNAs function as part of the RNA-induced silencing complex (RISC). Base-pairing between a seed region in the 5′ of a miRNA and the 3′ UTR of an mRNA guides RISC to target transcripts, which are then degraded, destabilized or translationally inhibited [7] . miRNA-mediated gene expression silencing has previously been shown to be important for a variety of physiological and pathological processes, such as developmental patterning, cancer progression, neuronal functions and dysfunctions [8] . Importantly, miRNAs are known for their rapid evolutionary dynamics, with dozens of novel miRNAs emerged in the genomes of individual species of nematode [9] , flies [10] . Novel miRNA emergence could affect expression of hundreds of genes, thus accelerating species-specific gene expression evolution. Identification of human-specific miRNAs To identify miRNAs specific to the human genome, we searched for orthologs of all 1,733 annotated mature human miRNAs (miRBase [11] version 17) in the genomes of 11 species: chimpanzee, gorilla, orangutan, rhesus macaque, marmoset, mouse, rat, dog, cow, opossum and chicken. To do so, we mapped miRNA precursors to each genome using reciprocal BLAST [12] or reciprocal LiftOver [13] . For 1,412 out of 1,426 annotated human miRNA precursors (99%) there was at least one ortholog in at least one species ( Supplementary Data 1 ). We next extracted mature miRNA orthologs from the precursor sequence alignment made using the Muscle sequence alignment algorithm [14] . On the basis of these data, we identified 10 mature human miRNAs with no detectable orthologs in any of the 11 species and 12 mature miRNAs with sequence changes in seed region that took place in the human lineage after the split with chimpanzee ( Supplementary Table S1 ). Expression pattern of human-specific miRNAs To estimate functional roles of newly emerged or newly mutated human miRNAs, we examined expression levels of these miRNAs in two brain regions, the prefrontal cortex and the cerebellum, of humans, chimpanzees and rhesus macaques using high-throughput RNA sequencing (RNA-seq). In agreement with previous observations in flies [10] , more ancient miRNAs, such as those conserved among mammals, tended to have higher expression levels than more recently emerged miRNAs, such as primate-specific miRNAs ( Fig. 1a,b ). Accordingly, all but one human-specific miRNA were expressed at extremely low levels in the human brain or not expressed at all ( Fig. 1a,b ). The only exception was miR-941. In both brain regions it was expressed higher than other human-specific or primate-specific miRNAs. Furthermore, miR-941 expression in the brain was comparable to the median level of conserved mammalian miRNAs ( Fig. 1a,b ). No miR-941 expression was observed in brains of chimpanzees and macaques. 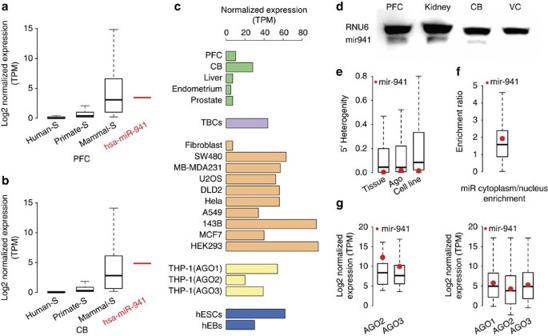Figure 1: miR-941 expression features. Expression levels of miR-941 and other human-specific miRNA, primate-specific miRNA and miRNA conserved among mammals in the human prefrontal cortex (a) and cerebellum (b). Expression of miR-941 in human tissues (green), human tonsillar B-cell populations (TBCs) (purple), human cell lines (orange), AGO co-immunoprecipitations in THP-1 cells (yellow) and human ESC and EB cells (blue) (c). miR-941 expression levels were estimated based on RNA-Seq data as Transcripts Per Million reads (TPM): number of reads mapped to the transcript normalized by the number of total mapped reads. Northern blot analysis of miR-941 expression in human prefrontal cortex (PFC), kidney, cerebellum (CB) and visual cortex (VC). U6 RNA (RNU6) was used as a loading control (d). Sequence heterogeneity of 5′ termini of miR-941 and other human miRNA. Lower sequence heterogeneity corresponds to a more defined seed region sequence, characteristic of functional miRNA (e). Cytoplasmic enrichment of miR-941 and other human miRNA in THP-1 cells. Enrichment of mature miRNA in the cytoplasm rather than in the nucleus is characteristic of the majority of functional miRNA (f). Co-immunoprecipitation with AGO proteins of miR-941 and other human miRNA in THP-1 cells (right panel) and Jurkat cells (left panel). Association with AGO proteins, the key components of the RISC complex, is characteristic of functional miRNA (g). Figure 1: miR-941 expression features. Expression levels of miR-941 and other human-specific miRNA, primate-specific miRNA and miRNA conserved among mammals in the human prefrontal cortex ( a ) and cerebellum ( b ). Expression of miR-941 in human tissues (green), human tonsillar B-cell populations (TBCs) (purple), human cell lines (orange), AGO co-immunoprecipitations in THP-1 cells (yellow) and human ESC and EB cells (blue) ( c ). miR-941 expression levels were estimated based on RNA-Seq data as Transcripts Per Million reads (TPM): number of reads mapped to the transcript normalized by the number of total mapped reads. Northern blot analysis of miR-941 expression in human prefrontal cortex (PFC), kidney, cerebellum (CB) and visual cortex (VC). U6 RNA (RNU6) was used as a loading control ( d ). Sequence heterogeneity of 5′ termini of miR-941 and other human miRNA. Lower sequence heterogeneity corresponds to a more defined seed region sequence, characteristic of functional miRNA ( e ). Cytoplasmic enrichment of miR-941 and other human miRNA in THP-1 cells. Enrichment of mature miRNA in the cytoplasm rather than in the nucleus is characteristic of the majority of functional miRNA ( f ). Co-immunoprecipitation with AGO proteins of miR-941 and other human miRNA in THP-1 cells (right panel) and Jurkat cells (left panel). Association with AGO proteins, the key components of the RISC complex, is characteristic of functional miRNA ( g ). Full size image Using published RNA-seq data from 23 tissues and cell lines, we further assessed miR-941 expression across human tissues and cell lines to obtain information for its tissue specificity. Besides the prefrontal cortex and the cerebellum [6] , miR-941 was expressed in liver, prostate, endometrium and six human tonsillar B-cell populations [15] , [16] , [17] , as well as in a wide range of human cell lines [18] , [19] ( Fig. 1c ; Supplementary Table S2 ). Notably, miR-941 expression levels were substantially higher in cancer-derived cell lines and human embryonic stem cells (hESCs) than in normal tissues or differentiated hESCs (embryoid body cells) ( Fig. 1c ). Is miR-941 a bona fide miRNA? By conducting northern Blot experiments, we confirmed the presence of mature miR-941 in human prefrontal cortex, cerebellum and kidney ( Fig. 1d , see Methods). Further, our analysis of sequence variations in miR-941 reads indicated reduced heterogeneity of the mature miRNA 5′ terminus—a sequence feature associated with functional miRNA [20] ( Fig. 1e ). Using RNA-seq data from THP-1 (human acute monocytic leukaemia cell line) nucleus and cytoplasm [21] , we further found that miR-941, like most functional miRNAs, is enriched in the cytoplasm ( Fig. 1f ). Finally, miR-941 was associated with AGO proteins, the key components of the RISC complex, in multiple AGO immunoprecipitation experiments conducted using various sequencing platforms-454, Illumina and SOLiD-in a number of human cell lines: hESCs, hNSCs, THP-1 and Jurkat cells [22] , [23] , [24] ( Supplementary Table S2 , Fig. 1c,g ). Notably, miR-941 was associated with AGO proteins at levels compatible to or exceeding those observed for conserved functional miRNAs ( Fig. 1g ). Thus, miR-941 displays all features of a functional miRNA. miR-941 sequence evolution In humans, miR-941 resides in the first intron of the DNAJC5 gene in chr20 q13.33. According to miRBase annotation, this region contains three copies of pre-miR-941, all capable of forming canonical stable hairpin structures ( Fig. 2a ). Remapping miR-941 precursor sequences to the human reference genome, we found not three, but seven copies of putative pre-miR-941 ( Supplementary Fig. S1 ). Each of the seven precursor copies contained a stable hairpin structure including mature miR-941 and miR-941-star sequences ( Fig. 2b,c ). Mature miR-941 and miR-941-star sequences complement each other, leaving two-nucleotide overhangs—a feature indicative of processing by Drosha and Dicer enzymes [7] ( Fig. 2b ). Reads corresponding to miR-941 and miR-941-star sequences could be identified in human ( Fig. 2c ), but not in chimpanzee or rhesus macaque RNA-seq data. 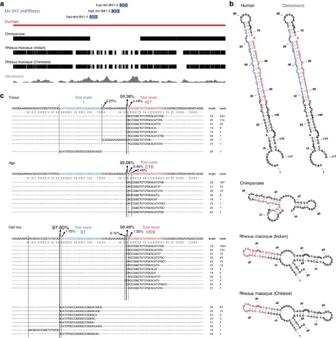Figure 2: miR-941 sequence evolution. Alignment of the genomic regions containing miR-941 precursors between the human, chimpanzee, rhesus macaque (Indian and Chinese) and Denisova genome (a). For the Denisova genome, sequence read coverage is shown. miR-941 precursor locations in the human genome are drawn based on the miRBase annotation. Secondary structure of transcripts corresponding to the miR-941 precursor sequence from the human, Denisova, chimpanzee, rhesus macaque (Indian and Chinese) genomes (b). Locations of the mature miR-941 (red) and miR-941-star (blue) sequences in the human precursor sequence and their corresponding locations in the other species' precursors are shown. RNA-seq read coverage of the mature miR-941 (red) and miR-941-star (blue) in human tissues (prefrontal cortex and cerebellum), AGO co-immunoprecipitations experiments and human cell lines (c). The complete list of data sets used is listed inSupplementary Table S3. Figure 2: miR-941 sequence evolution. Alignment of the genomic regions containing miR-941 precursors between the human, chimpanzee, rhesus macaque (Indian and Chinese) and Denisova genome ( a ). For the Denisova genome, sequence read coverage is shown. miR-941 precursor locations in the human genome are drawn based on the miRBase annotation. Secondary structure of transcripts corresponding to the miR-941 precursor sequence from the human, Denisova, chimpanzee, rhesus macaque (Indian and Chinese) genomes ( b ). Locations of the mature miR-941 (red) and miR-941-star (blue) sequences in the human precursor sequence and their corresponding locations in the other species' precursors are shown. RNA-seq read coverage of the mature miR-941 (red) and miR-941-star (blue) in human tissues (prefrontal cortex and cerebellum), AGO co-immunoprecipitations experiments and human cell lines ( c ). The complete list of data sets used is listed in Supplementary Table S3 . Full size image In the human and macaque genomes, the miR-941 precursor region are composed of tandem repeats displaying greater interspecies than intraspecies variation, indicating rapid locus evolution ( Supplementary Fig. S2a-e ). Correspondingly, almost the entire repeat region is lost in the chimpanzee genome ( Fig. 2a ). One of the repeat copies present in the macaque genome differs from the rest and more closely resembles the human variant of the tandem repeats. It is therefore likely that tandem repeats present in the human genome were derived from this repeat variant, which has undergone copy number expansion and replaced other repeat variants in the human lineage ( Supplementary Fig. S2f ). It takes two copies of the human version of tandem repeats to form pre-miR-941, with the apex of the precursor stem loop structure coinciding with the boundary between repeats ( Supplementary Fig. S2g ). As a consequence, corresponding genomic regions in chimpanzees and macaque could not form stable miRNA precursor hairpins ( Fig. 2a,b ). To confirm the validity of the reference genome sequences, we amplified and sequenced the pre-miR-941 locus in one human, eight chimpanzees and six rhesus macaques ( Supplementary Table S3 ). The sequences matched the reference genome sequences ( Supplementary Fig. S3 ). These results demonstrate that miR-941 precursor sequence has evolved in humans, most likely after the human–chimpanzee split, through tandem repeat replacement and expansion. To obtain more precise estimates of the miR-941 precursor emergence in the human evolutionary lineage, we examined the genome of Denisova—an extinct hominid species that diverged from the human lineage approximately one million years ago. Although overall genome sequencing coverage was relatively low (1.9-fold), we found that the corresponding genomic locus in the Denisova genome contains at least two copies of the miR-941 precursor sequence ( Fig. 2a , see Methods). Thus, pre-miR-941 formation, as well as copy-number increase, took place between the chimpanzee and the Denisova bifurcations: between six to seven million and one million years ago ( Fig. 3a ). 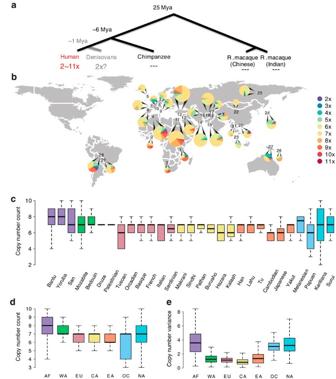Figure 3: miR-941 sequence copy number variation among human populations. Phylogenetic tree showing miR-941 precursor copy numbers in humans, Denisova, chimpanzees and rhesus macaques (a). Distribution of miR-941 copy numbers in human populations from the HGDP-CEPH Human Genome Diversity Cell Line Panel (b). Each circle represents a population, circle size is proportional to the number chromosomes sampled, colours represent proportions of copy miR-941 precursor copy numbers in each population. The number next to each circle indicates population identity, as listed inSupplementary Table S7. Average miR-941 precursor copy numbers differences among populations (c) as well as geographical regions (d). miR-941 copy number variation among geographical regions (e). Variation of the average copy number estimates and variation estimates was calculating by bootstrapping sequenced precursor loci 1,000 times. The labels indicate: AF: Africans, WA: Western Asians, EU: Europeans, CA: central and Southern Asians, EA: Eastern Asians, OC: Oceanians, NA: native Americans. Figure 3: miR-941 sequence copy number variation among human populations. Phylogenetic tree showing miR-941 precursor copy numbers in humans, Denisova, chimpanzees and rhesus macaques ( a ). Distribution of miR-941 copy numbers in human populations from the HGDP-CEPH Human Genome Diversity Cell Line Panel ( b ). Each circle represents a population, circle size is proportional to the number chromosomes sampled, colours represent proportions of copy miR-941 precursor copy numbers in each population. The number next to each circle indicates population identity, as listed in Supplementary Table S7 . Average miR-941 precursor copy numbers differences among populations ( c ) as well as geographical regions ( d ). miR-941 copy number variation among geographical regions ( e ). Variation of the average copy number estimates and variation estimates was calculating by bootstrapping sequenced precursor loci 1,000 times. The labels indicate: AF: Africans, WA: Western Asians, EU: Europeans, CA: central and Southern Asians, EA: Eastern Asians, OC: Oceanians, NA: native Americans. Full size image Interestingly, pre-miR-941 copy number might continue to change after human and Denisova split. In the human genome, pre-miR-941 is located in a genomic region displaying copy-number variation among four contemporary human populations: Yoruba, Caucasian, Chinese and Japanese [25] . This is not unexpected, given general instability of genomic regions formed by tandem repeats. To examine this further, we amplified and sequenced the pre-miR-941 locus in 558 individuals from 38 populations from the HGDP-CEPH Human Genome Diversity Cell Line Panel [26] . We found a large degree of variation in pre-miR-941 copy number among contemporary humans, ranging from 2 to 11 copies ( Fig. 3b ). This variation was not caused by PCR amplification artifacts, as indicated by replicate amplifications from six individuals of African descent. Further, both pre-miR-941 copy number and copy-number variation differed significantly among populations from different geographical regions (Kruskal–Wallis test for copy number difference, P =0.000065, Bartlett's test and Levene's test for copy number variation difference, P <0.000073). The average pre-miR-941 copy number decreased from the west to the east: from eight copies in sub-Saharan Africans to six copies in Eastern Asians ( Fig. 3c,d ). miR-941 precursor copy number variation was also significantly higher in sub-Saharan Africans compared with 'out of Africa' populations, with the exception of Oceanians and native Americans (Bartlett's test, P =0.00064, Levene's test, P =0.00078) ( Fig. 3e ). Identification of miR-941 target genes The seed sequence of miR-941 differs from seed sequences of other human miRNAs, suggesting specific regulatory effects. To identify potential targets and potential functions of miR-941, we transfected three human cell lines, 293T, HEK and HSF2, with miR-941 duplex or mock duplex. We then measured gene expression changes in each cell line 24 h after transfection, using Affymetrix Human Genome U133 Plus 2.0 microarrays. In all three cell lines, we observed significant overrepresentation of gene expression inhibition among miR-941 targets predicted by TargetScan [27] or other five miRNA target prediction algorithms [28] , [29] , [30] , [31] , [32] ( Fig. 4a-c ; Supplementary Fig. S4 and Supplementary Table S4 ). Because of the evolutionary novelty of miR-941, target site conservation was not required during the target prediction. 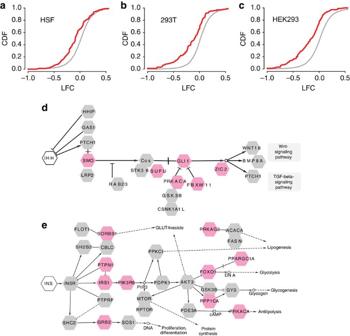Figure 4: miRNA-941 targets identification and functional analysis. Cumulative distribution plots of log2-transformed gene expression fold-changes (LFC) for genes containing miR-941 target sites predicted by TargetScan (red) and all other expressed genes (grey) after transfection with miR-941 duplex or mock duplex in the three human cells lines: HSF (a), 293T (b) and HEK (c). Prevalence of the negative LFC measurements among predicted miR-941 targets indicates inhibitory effect of miR-941 duplex transfection, the y axis shows cumulative distribution function (CDF) of LFC distribution. Experimentally verified miR-941 target genes (pink) in hedgehog signalling pathway (d) and insulin signalling pathway (e). Figure 4: miRNA-941 targets identification and functional analysis. Cumulative distribution plots of log2-transformed gene expression fold-changes (LFC) for genes containing miR-941 target sites predicted by TargetScan (red) and all other expressed genes (grey) after transfection with miR-941 duplex or mock duplex in the three human cells lines: HSF ( a ), 293T ( b ) and HEK ( c ). Prevalence of the negative LFC measurements among predicted miR-941 targets indicates inhibitory effect of miR-941 duplex transfection, the y axis shows cumulative distribution function (CDF) of LFC distribution. Experimentally verified miR-941 target genes (pink) in hedgehog signalling pathway ( d ) and insulin signalling pathway ( e ). Full size image We then classified predicted miR-941 targets downregulated after transfection with miR-941 duplex, but not the negative control, in all three human cell lines, as experimentally verified miR-941 target genes ( Supplementary Data 2 , see Methods). Compared with other genes expressed in the cell lines, experimentally verified miR-941 target genes showed significant enrichment in two KEGG pathways: hedgehog-signalling pathway and insulin-signalling pathway (hypergeometric test, Bonferroni corrected P <0.032). Notably, in both pathways, miR-941 targets some of the key annotated pathway components, including SMO, SUFU and GLI1 in the hedgehog-signalling pathway [33] and IRS1, PPARGC1A and FOXO1 in the insulin-signalling pathway [34] ( Fig. 4d,f ). To further test whether these experimentally verified miR-941 targets represent direct targets of miR-941, immunoprecipitation by Ago2 (Ago2-IP) was conducted in the human 293T cell line. We then used Affymetrix microarrays to compare concentrations of transcripts captured in Ago2-IP in cells overexpressing miR-941 and in negative controls. We found that genes containing predicted miR-941-binding sites and enriched in Ago2-IP in cells overexpressing miR-941, showed significant downregulation in miR-941 transfection experiments ( Supplementary Fig. S5a and Supplementary Data 2 ). Repeating our analyses based on these targets we confirmed significant enrichment of these Genes in insulin signalling pathway (hypergeometric test, Bonferroni corrected P =0.041). Evolution of miRNA-941-guided regulation The emergence of miR-941 in humans might have led to the downregulation of genes containing corresponding binding sites in their 3′ UTRs. To test this, we examined expression of miR-941 target genes in human, chimpanzee and rhesus macaque brains. mRNA expression was measured in the prefrontal cortex of five human, five chimpanzee and two rhesus macaque adult individuals and in the cerebellum of five human, five chimpanzee and one rhesus macaque adult individuals using Affymetrix Gene1.0 ST arrays [6] . Using macaque as an out-group, we assigned expression changes to either the human or the chimpanzee lineages assuming maximum parsimony. For miR-941 target genes verified by miR-941 transfection, we found a significant excess of transcriptional inhibition in the human but not the chimpanzee lineage (Binomial test, P <0.004, Fig. 5a ; Supplementary Table S5 and Supplementary Data 2 ). The excess of transcriptional inhibition in the human linage could also be observed using putative direct miR-941 target genes identified in Ago2-IP ( Supplementary Data 2 and Supplementary Fig. 5b ). Further, the inhibitory effects of miR-941 in the human brain largely overlapped between the two brain regions (binomial test, P =0.0000045). Notably, among the miR-941 target genes showing human-specific downregulation in both brain regions is the host gene of miR-941, DNAJC5 , containing three candidate miR-941-binding sites in its 3′ UTR. 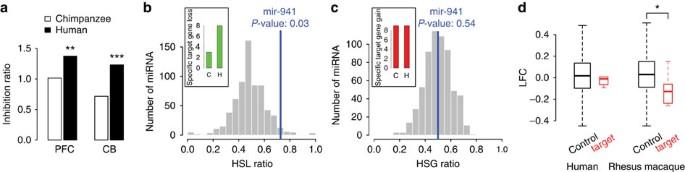Figure 5: Evolution of miRNA-941-guided regulation. Transcriptional inhibition of experimentally verified miR-941 target genes in the prefrontal cortex (PFC) and cerebellum (CB) (a). Inhibition ratio was calculated as the ratio between the numbers of experimentally verified miR-941 target genes showing lineage-specific expression decrease and not showing such as a decrease on the human (black) and the chimpanzee (white) evolutionary lineages. The proportions of experimentally verified miR-941 target genes, showing lineage-specific expression decrease on the human and the chimpanzee lineages were compared using Binomial test. The asterisks show significance of transcriptional inhibition excess on the human lineage (*P<0.05, **P<0.01, ***P<0.001). Human-specific loss (HSL) (b) and human-specific gain (HSG) (c) of binding sites for miR-941 (blue) and for all annotated human miRNA conserved between humans, chimpanzees and macaques (grey). The inserts show numbers of miR-941 target gene gains (red) and losses (green) on the human and the chimpanzee evolutionary lineages. Regulatory effect of miR-941 on genes containing miR-941-binding sites lost on the human evolutionary lineage (d). Genes containing miR-941 predicted binding sites in the rhesus macaque and chimpanzee genomes, but not in the human genome, (red) were significantly downregulated compared with non-target genes (black) after miR-941 transfection in the three macaque cell lines (one-sided Wilcoxon signed-rank test,P=0.042) (right), but not in the three human cell lines (one-sided Wilcoxon signed-rank test,P=0.46) (left). The y axis shows log2-transformed gene expression fold-changes (LFC) in the cell lines after transfection. Figure 5: Evolution of miRNA-941-guided regulation. Transcriptional inhibition of experimentally verified miR-941 target genes in the prefrontal cortex (PFC) and cerebellum (CB) ( a ). Inhibition ratio was calculated as the ratio between the numbers of experimentally verified miR-941 target genes showing lineage-specific expression decrease and not showing such as a decrease on the human (black) and the chimpanzee (white) evolutionary lineages. The proportions of experimentally verified miR-941 target genes, showing lineage-specific expression decrease on the human and the chimpanzee lineages were compared using Binomial test. The asterisks show significance of transcriptional inhibition excess on the human lineage (* P <0.05, ** P <0.01, *** P <0.001). Human-specific loss (HSL) ( b ) and human-specific gain (HSG) ( c ) of binding sites for miR-941 (blue) and for all annotated human miRNA conserved between humans, chimpanzees and macaques (grey). The inserts show numbers of miR-941 target gene gains (red) and losses (green) on the human and the chimpanzee evolutionary lineages. Regulatory effect of miR-941 on genes containing miR-941-binding sites lost on the human evolutionary lineage ( d ). Genes containing miR-941 predicted binding sites in the rhesus macaque and chimpanzee genomes, but not in the human genome, (red) were significantly downregulated compared with non-target genes (black) after miR-941 transfection in the three macaque cell lines (one-sided Wilcoxon signed-rank test, P =0.042) (right), but not in the three human cell lines (one-sided Wilcoxon signed-rank test, P =0.46) (left). The y axis shows log2-transformed gene expression fold-changes (LFC) in the cell lines after transfection. Full size image Taken together, our results demonstrate that miR-941 is highly expressed compared with other newly emerged human-specific miRNA in the prefrontal cortex and cerebellum, as well as in multiple human cell lines, and has detectable regulatory effects on gene expression in the human brain. Although some of these regulatory effects might be beneficial, introduction of a new miRNA into an established regulatory network might also result in deleterious expression changes. In this case, natural selection would lead to rapid elimination either of miRNA-941 itself or of miR-941-binding sites responsible for deleterious regulatory effects. As miR-941 was not eliminated, we predict that more miR-941-binding sites would be lost in the human than in the chimpanzee lineage, as the latter was not exposed to miR-941 expression. Using macaque as an outgroup, we indeed found greater loss of predicted miR-941-binding sites in human than in chimpanzee. Specifically, eight miR-941-binding sites were lost in the human lineage and three in the chimpanzee lineage ( Fig. 5b ; Supplementary Table S6 , see Methods). Compared with the predicted loss of binding sites based on all annotated miRNAs present in the human, chimpanzee and rhesus macaque genomes, this excessive loss of miR-941 sites is not expected to occur by chance ( P =0.03, Fig. 5b ). In contrast, we observed no difference in miR-941-binding site gains between human and chimpanzee ( P =0.54, Fig. 5c ). Although these results are based on predicted miRNA-binding sites, we set out to test them further using experimentally verified targets of miR-941. We transfected two macaque kidney cell lines (LLCMK2 and FrhK-4) and one macaque skin fibroblast cell line with miR-941 duplex or a mock duplex. We then measured gene expression changes in each cell line 24 h after the transfection using microarrays. In all three cell lines we observed significant overrepresentation of gene expression inhibition among miR-941 targets predicted by TargetScan (Kolmogorov–Smirnov test, P <0.000037) ( Supplementary Fig. S6 ). Furthermore, for genes containing miR-941 targets sites in both macaques and humans, there was a significant overlap of experimentally verified miR-941 targets between human and macaque transfection experiments (binomial test, P= 0.0027). Importantly, genes containing predicted miR-941-binding sites in rhesus macaque and chimpanzee, but not in human, were significantly downregulated in the three macaque cell lines upon miR-941 transfection ( P =0.042), but not in the three human cell lines ( P =0.46) ( Fig. 5d ). Furthermore, genes that lost miR-941 target sites in the human lineage were significantly overrepresented among miR-941 targets experimentally verified in the three macaque cell lines ( P =0.036). Taken together, these results show that miR-941 emergence and copy number increase in the human lineage indeed resulted in accelerated loss of miR-941-binding sites. miRNA-induced downregulation could be avoided by other mechanisms that do not involve binding sites loss, such as competitive binding of RNA-binding proteins preventing target incorporation into the RISC complex [35] . To test whether any putative miR-941 targets might avoid downregulation by such indirect mechanisms, we looked for genes showing downregulation in miR-941 transfection experiments in rhesus macaque cell lines, but not in human cell lines. We identified 49 genes that contained miR-941-binding sites in both the human and the macaque genomes and showed no detectable downregulation after miR-941 transfection in the three human cell lines. Out of these 49 genes, 19 were downregulated after miR-941 transfection in macaque cell lines. Testing the abundance of these 19 genes in Ago2-IP conducted in human cells, we found significant under-representation of these transcripts in Ago2-IP compared with other predicted miR-941 target genes expressed in the brain (Wilcoxon signed-rank test, P =0.00067) ( Supplementary Fig. S7 ). This result indicates that some of the predicted miR-941 targets might avoid downregulation by escaping incorporation into the RISC complex. miRNAs are powerful gene expression regulators targeting most human genes [36] . Accordingly, birth of a novel miRNA might influence expression of hundreds of genes. Although some of these gene expression changes might be beneficial, most would be expected to be deleterious, an observation that has been experimentally verified in fly [37] . At the same time, novel miRNAs were shown to emerge at a relatively rapid rate, either by appearance of transcribed hairpin structures or by mutations in the miRNA seed region [10] , With one exception found in flies [10] , this limits deleterious effects of their emergence on transcriptome regulation. With time most novel miRNAs disappear, few being incorporated into regulatory networks and gradually increasing their expression level [38] . This trend can be also clearly observed in our data with one notable exception of miR-941. Although miR-941 precursor sequence has evolved after separation of the human and the chimpanzee lineages that took place as recently as 6–7 million years ago, expression level of miR-941 in the human brain is high and comparable to expression levels of functional miRNAs conserved in mammals. We speculate that the high miR-941 expression level is at least partially owing to amplification of its precursor sequence in the human lineage. The genome of Denisova, the extinct human relatives that split from the human lineage approximately one million years ago already contained at least two copies of miR-941 precursor. Genomes of contemporary humans contain 2–11 copies of miR-941 precursor, with an average of 8 copies found in sub-Samarian Africa, an average of 7 copies in Europe, America, Oceania and most of Asia, and an average of 6 copies in East Asia. One of the tandem repeats constituting pre-miR-941 in humans contains a C to G substitution at position 15 of the mature sequence. Mature miRNA sequences containing this mutation could be readily detected in human tissues, cell lines and AGO immunoprecipitation experiments, along with the wild-type miR-941 sequence, in ~15–85% ratio. This shows that both mutant and wild-type versions of pre-miR-941 are expressed in humans and indicates that multiple copies of wild-type pre-miR-941 could be transcriptionally active. In this study, however, we did not investigate whether pre-miR-941 copy number correlates with expression level of miR-941 in human tissues or cell lines. Rapid increase in the expression of a novel miRNA is predicted to result in deleterious regulatory effects. In agreement with this notion, we observed accelerated loss of miR-941-binding sites in the human lineage. Notably, miR-941-binding sites lost in humans were targeted by miR-941 transfection into macaque cell lines. This confirms that emergence of miR-941 in the human lineage would affect expression of genes, which accidentally contain these binding sites. Given the extraordinarily high miR-941 expression in humans, it is appealing to speculate that beneficial effects of miR-941 emergence offset deleterious ones. miR-941 transfection into human cell lines preferentially affected genes in two pathways: hedgehog signalling and insulin signalling. Notably, in both pathways, miR-941 targeted some of the key components ( Fig. 4d,f ). The hedgehog-signaling pathway has a central role in embryonic development and is involved in the maintenance of stem cell populations in adults [33] . Abnormal activation of this pathway was further observed in certain forms of cancer [33] . It is, therefore of interest that miR-941 expression was highest in hESCs and in many cancer-derived human cell lines, and decreased upon stem cell differentiation. Humans display both increased longevity and increased occurrence of certain forms of cancer compared with both chimpanzees and macaques [39] . It is, therefore, appealing to speculate that emergence of miR-941 enhanced the maintenance of adult stem cell populations, thus supporting longer human lifespan, but rendering human cells more prone to malignant transformation. The role of miR-941 in the regulation of insulin signaling adds support to this notion. The insulin-signaling pathway was consistently implicated in lifespan regulation in many species, including humans. Notably, experimentally verified targets of miR-941 within this pathway include genes directly shown to be involved in lifespan extension in model organisms: IRS1, PPARGC1A and FOXO1 [40] (ref. 40). Furthermore, FOXO1 was linked to extended human longevity [41] . Previous studies have shown that intronic miRNAs are usually transcribed along with their host genes and could exert synergistic and antagonistic regulatory effects on their host genes [42] . It is, therefore, notable that the host gene of miR-941, DNAJC5 , shows human-specific downregulation in both brain regions. DNAJC5 encodes cysteine-string protein-α (CSPα). CSPα resides in presynaptic terminals, clathrin-coated vesicles and neuroendocrine secretory granules and is involved in neurotransmitter release [43] , [44] , [45] and is mainly expressed in neurons, rather than glia [46] , [47] , [48] , [49] . Deletion of CSPα in flies and mice impairs synaptic function and results in neurodegeneration, behavioural deficits and premature death [45] , [50] . Furthermore, CSPα has been linked to Huntington's and Parkinson's disease, as well as adult neuronal neroid-lipofuscinosis, a common inherited neurodegenerative disease [45] , [51] , [52] . By querying a protein–protein interaction database, seven genes show direct interaction with CSPα. Two out of these seven genes, PRKACA and RAB3A , are among the experimentally verified miR-941 targets showing human-specific downregulation in brain. Similar to CSPα, RAB3A also functions in neurotransmitter release [53] . Furthermore, WDR7 , an interaction partner of RAB3A , similarly involved in the control of calcium-dependent neurotransmitter release [54] , is also the among experimentally verified miR-941 target genes showing human-specific downregulation. Another hint for the potential involvement of miR-941 and its host gene in neuronal functions comes from studies of a microdeletion in chr20 q13.33 chromosomal region containing pre-miR-941. Individuals containing this microdeletion display mental retardation, developmental delay, as well as speech and language defects [55] . Besides the pre-miR-941 cluster, the deleted region usually contains more than 20 protein-coding genes. Still, it remains possible that miR-941 might be responsible for or contribute to the disease phenotype. In conclusion, we show that the emergence and rapid expansion of miR-941 precursor sequence took place in the human evolutionary lineage between six and one million years ago, and was accompanied by an exceptional increase in miR-941 expression level. The emergence of miR-941 was accompanied by accelerated loss of its binding sites, presumably due to deleterious effects of miR-941-guided regulation. Functionally, miR-941 could be associated with hedgehog- and insulin-signaling pathways, and thus potentially has a role in the evolution of human longevity. Furthermore, human-specific effects of miR-941 regulation are detectable in the human brain and affect genes involved in neurotransmitter signaling. Deletion of the genomic region containing pre-miR-941 results in disruption of human-specific cognitive functions including language and speech. Taken together, the unusual features of miR-941 evolution, as well as its potential association with functions linked to human longevity and cognition, suggest roles of miR-941 in the evolution of human-specific phenotypes. More generally, miR-941 evolution provides an example for rapid emergence of a novel post-transcriptional regulator, thus allowing for a rare opportunity to study consequences of this process on evolution of a regulatory network. Ethics statement Informed consent for the use of human tissues for research was obtained in writing from all donors or their next of kin. All non-human primates used in this study suffered sudden deaths for reasons other than their participation in this study and without any relation to the tissue used. Biomedical Research Ethics Committee of Shanghai Institutes for Biological Sciences completed the review of the use and care of the animals in the research project (approval ID: ER-SIBS-260802P). Human-specific miRNA identification Human miRNA annotations were downloaded from miRBase [11] (version 17). To identify human-specific miRNA, orthologs of all annotated human miRNA precursors were detected using reciprocal BLAST [12] or reciprocal LiftOver [13] with default settings and required the length of hit sequence to be >60% and <130% of query sequence in the genomes of 11 species: chimpanzee (UCSC genome accession code: panTro3), gorilla (UCSC genome accession code: gorGor3), orangutan (UCSC genome accession code: ponAbe2), rhesus macaque (UCSC genome accession code: rheMac2), marmoset (UCSC genome accession code: calJac3), mouse (UCSC genome accession code: mm9), rat (UCSC genome accession code: rn4), dog (UCSC genome accession code: canFam2), cow (UCSC genome accession code: bosTau6), opossum (UCSC genome accession code: monDom5) and chicken (UCSC genome accession code: galGal3). Mature miRNA sequences were further extracted from precursor sequence alignment using muscle [14] ( Supplementary Data 1 ). The genome sequences of human and the other 11 species were downloaded from UCSC [13] . Human-specific miRNA were classified as miRNA with not detectable orthologs in any of the 11 species or with sequence changes in the seed region that took place on the human evolutionary lineage after the split with chimpanzee ( Supplementary Table S1 ). Expression pattern of miR-941 miR-941 expression across human tissues, cell lines and multiple AGO immunoprecipitation experiments were estimated using the following published RNA-seq data sets: prefrontal cortex and cerebellum [6] , liver [15] , endometrium [16] , six human tonsillar B-cell populations [17] , human cell lines [18] , [19] AGO immunoprecipitation experiments [22] , [23] , [24] ( Supplementary Table S2 ). miRNA 5′ heterogeneity and cytoplasm/nucleus enrichment analysis miRNA 5′ heterogeneity was estimated as described elsewhere [20] . Cytoplasm/nucleus enrichment analysis of miR-941 mature sequence was based on the data from THP-1 (Human acute monocytic leukaemia cell line) as described in [21] ref. 21. More detailed method descriptions were in Supplementary Methods . miRNA-941 sequence evolution analysis Number of miR-941 precursors in the reference human genome was estimated by mapping annotated miR-941 precursor sequences to the genome (UCSC genome accession code hg19) using BLAST or BLAT. RNA secondary structures of the human miR-941 precursor and corresponding regions in the genomes of chimpanzee, Indian and Chinese rhesus macaques and Denisova were analysed by RNA-fold [56] . Genomic locations of miR-941 mature sequence and miR-941-star sequence were determined by mapping RNA-seq reads to the miR-941 precursor sequence. Number of miR-941 precursors in Denisova was estimated by mapping publicly available Denisova sequence reads to the human reference genome. More detailed method descriptions were in Supplementary Methods. To determine miR-941 precursor copy number in humans and verify its absence in the chimpanzee and rhesus macaque genomes, we amplified and sequenced the miR-941 genomic locus from the genomes of one human, eight chimpanzee and six rhesus macaque individuals. Sample and primer information used in this analysis is listed in Supplementary Table S3 . miR-941 precursor copy number variation analysis To determine miR-941 precursor copy number variation among human populations we amplified and sequenced genomic region containing miR-941 precursor sequences in 558 individuals from 38 populations of the HGDP-CEPH Human Genome Diversity Cell Line Panel [26] ( Supplementary Table S7 ). More detailed PCR method description was in the Supplementary Methods . miR-941 precursor copy number was estimated by mapping annotated miR-941 precursor sequences to the amplified and sequenced genomic regions using Blat. The miR-941 precursor copy number variation results were robust to use of other copy number quantification procedures: merging overlapped precursors or counting numbers of tandem repeats constituting miR-941 precursor. miR-941 precursor copy number difference among populations from different geographical regions was tested by Kruskal–Wallis test. miR-941 precursor copy number variant difference among populations from different geographical regions and between sub-Saharan Africans and 'out of Africa' populations were tested by Bartlett's test and Levene's test. Mozabite population was classified as 'West Asians' rather than 'Africans' in the region-based copy number and copy number variation analyses. To confirm the robustness of miR-941 precursor copy number estimates among humans obtained using PCR, we did repeat PCR amplification followed by sequencing for six individuals from African populations. In all six cases, miR-941 precursor copy number estimates agreed between the experimental replicates (see Supplementary Fig. S8 ). miRNA transfection, microarray data analysis and mir-941 target effects miRNA transfection experiments were conducted in six cell lines—two human derived kidney cell lines (HEK and 293T), one human skin fibroblast cell line (HSF2), two macaque derived kidney cell lines (LLCMK2 and FrhK-4), one macaque skin fibroblast cell line—as described previously in [6] ref. 6. R RMA package was used to quantify gene expression levels. Ago2 immunoprecipitation (Ago2-IP) experiments after miR-941 overexpression were conducted in 293T cell line. Briefly, all transfections were performed using human 293T cells cultured in 6-well tissue culture plates. Lipofectamine 2,000 (Invitrogen) was used for a Synthetic miR-941 or a scrambled oligo transfection, at 30 nmol l −1 each (final concentration) per 1×10 6 cells per well of a six-well plate using DharmaFECT (GE Healthcare). Total 5×10 6 cells were collected and subjected to Ago2 immunoprecipitation (Ago2-IP) using the RNA isolation kit Mouse Ago2 (Wako Chemicals) according to the manufacturer's instructions. For a negative control, immunoprecipitation was performed using non-immune IgG beads prepared with the antibody immobilization bead kit (Wako Chemicals). The IP pull down RNA was used as template for an ' in vitro ' transcription reaction generating biotin-labeled antisense cRNA. The cRNA was analysed on Affymetrix Human Genome U133 Plus 2.0 arrays following the manufacturer's instructions. The R RMA package was used to quantify gene expression levels. We used GOstats [57] to investigate putative functions of experimentally verified target genes of miR-941 in human cell lines based on our transfection results. More detailed method descriptions were in the Supplementary Methods . Affymetrix exon array experiment Cerebellum mRNA samples from five human, five chimpanzee and one rhesus macaque for Affymetrix Human Exon 1.0. ST Arrays were prepared following the standard GeneChip Whole Transcript (WT) Sense Target Labelling Assay. We processed Exon Array data sets following the steps described in [6] ref. 6. mRNA samples from prefrontal cortex were downloaded from [6] . miRNA-941 northern blot Northern blot experiments were conducted in human prefrontal cortex, cerebellum, visual cortex and kidney. Briefly, 10 ng total RNA for each sample was analysed in 15% TBE-Urea pre-cast Gel (Invitrogen). RNAs were transferred onto positively charged hybond-N + nylon membrane (GE Healthcare Life Sciences) by a Semi-Dry Electrophoretic Transfer Cell (Bio-Rad). Oligonucleotide probes were 5′-end-labeled with [γ- 32 P] ATP using T4 polynucleotide kinase (NEB). The membranes were probed at 39 °C with the hybridization solution (Roche) overnight. The membranes were washed by 2× SSC and 0.5% SDS twice at 39 °C. Radioactive signals were quantified using Quantity ONE (Bio-Rad). The result shows miR-941 has on average 1.2-fold higher expression in the CB compared with PFC ( Supplementary Table S8 ). This result is in general agreement with RNA-seq measurements. Evolution of miRNA-941-guided regulation The approach to calculating miR-941 regulation effect on human-specific gene expression changing in prefrontal cortex and cerebellum was adopted and modified from [6] . More detailed method descriptions were in the Supplementary Methods . Species-specific gain/loss of miR-941 target sites was estimated using binding site predictions by TargetScan based on human, chimpanzee and rhesus macaque 3′ UTR sequence alignments. Specifically, 3′ UTR sequence alignments of human, chimpanzee and rhesus macaque were extracted from 3′ UTR sequence alignment file downloaded from TargetScan website [27] . Only the alignments with <5% of the gap sequence in human, chimpanzee and macaque were used for downstream analysis. TargetScan was used to predict miR-941 target sites across three species. Gain/loss of the target sites on the human and the chimpanzee lineages was calculated using rhesus macaque sequence as an outgroup. Human-specific gain (HSG) ratio of miR-941 target genes was calculated as the ratio between HSG miR-941 target gene number and the total number of target genes gained on the human and the chimpanzee lineages. Human-specific loss (HSL) ratio was calculated as the ratio between the number of HSL of miR-941 target genes and the total number of target genes lost on the human and the chimpanzee lineages. The genes shown interaction with CSPα are queried from STRING database, which contains known and redicted rotein interactions [58] . In total seven genes ( RAB3A, VAMP2 , VAMP7, SYT1, HSPA8, CFTR, PRKACA ) were returned using experiments and textmining methods plus medium confidence score (score >0.4) filtering. Accession codes: All original microarray data are deposited in the NCBI GEO database GSE35621 . How to cite this article : Hu, H.Y. et al . Evolution of the human-specific microRNA miR-941. Nat. Commun. 3:1145 doi: 10.1038/ncomms2146 (2012).